Classification of stable three-dimensional Dirac semimetals with nontrivial topology A three-dimensional (3D) Dirac semimetal (SM) is the 3D analogue of graphene having linear energy dispersion around Fermi points. Owing to the nontrivial topology of electronic wave functions, the 3D Dirac SM shows nontrivial physical properties and hosts various exotic quantum states such as Weyl SMs and topological insulators under proper external conditions. There are several kinds of Dirac SMs proposed theoretically and partly confirmed experimentally, but its unified picture is still missing. Here we propose a general framework to classify stable 3D Dirac SMs in systems having the time-reversal, inversion and uniaxial rotational symmetries. We show that there are two distinct classes of 3D Dirac SMs. In one class, the Dirac SM possesses a single Dirac point (DP) at a time-reversal invariant momentum on the rotation axis. Whereas the other class of Dirac SMs have a pair of DPs created by band inversion, and carry a quantized topological invariant. A Dirac semimetal (SM) indicates a phase whose low-energy excitations can be described by pseudorelativistic Dirac fermions with linear energy dispersion. Before the discovery of three-dimensional (3D) topological insulators [1] , [2] , graphene [3] has been considered as the unique system where the intriguing properties of two-dimensional (2D) Dirac fermions can be observed. However, the recent progress in the field of topological insulators has shown that stable 2D Dirac fermions exist ubiquitously on the surface of 3D topological insulators [1] , [2] . Moreover, through the careful studies on the topological phase transition between a 3D topological insulator and a normal insulator [4] , [5] , [6] , [7] , [8] , it is demonstrated that even the 3D Dirac fermions with the linear dispersion in all three momentum directions can be observed in the same material if we can reach the quantum critical point. As the 3D Dirac point (DP) with fourfold degeneracy does not carry a Chern number, the degeneracy at the gap-closing point can be easily lifted by small external perturbations, hence, the 3D Dirac fermions can be observed only at the single quantum critical point. However, the approach to the quantum critical point requires the intricate fine-tuning of the alloy chemical compositions [7] , [8] , which limits the accessibility to the fascinating physics of 3D Dirac fermions in experiments. The breakthrough in the search for stable 3D Dirac SMs is achieved in the recent series of studies on Na 3 Bi (refs 9 , 10 ) and Cd 3 As 2 (refs 11 , 12 , 13 , 14 ) compounds, where a pair of 3D DPs stably exist on the k z axis. The stability of the 3D DP in these materials stems from the fact that the system has additional crystalline symmetries other than the time-reversal symmetry (TRS) and inversion symmetry (IS) [15] , [16] , [17] , [18] , [19] , [20] . For instance, Young et al . [15] , [16] have proposed that particular space groups allow 3D DPs as symmetry protected degeneracies. Also, Wang et al . have shown the symmetry protection of the 3D DPs through the detailed symmetry analysis of Na 3 Bi (ref. 17 ) and Cd 3 As 2 (ref. 18 ). In the present paper, we propose a general framework to classify stable 3D Dirac SMs in systems with TRS, IS and uniaxial rotation symmetry, which are the most common symmetries of crystalline solids. Through the careful examination of the condition for the accidental band crossing (ABC), we have accomplished the complete classification of stable 3D Dirac SMs, and uncovered that there are two broad classes of 3D Dirac SMs. The Dirac SMs belonging to the first class are created via a band inversion, and have a pair of DPs on the rotation axis away from the time-reversal invariant momentum (TRIM). On the other hand, the second class of Dirac SMs have a single DP at a TRIM on the rotation axis where the band crossing is ensured by the lattice symmetry. In particular, we find that the first class of 3D Dirac SMs have nontrivial topological properties. We have clarified the fundamental relationship between the crystalline symmetries and the topological property of 3D Dirac SMs, and demonstrated that the 3D topological Dirac SM generally mediates the topological quantum phase transition between a normal insulator and a 3D weak topological insulator (or a topological crystalline insulator). In fact, the 3D topological Dirac SM itself is a parent state of 3D topological insulators, which turns into either a 3D strong topological insulator [17] , [18] or a 3D topological crystalline insulator when the 3D DP acquires a mass gap because of symmetry breaking. Basic principles to create 3D Dirac semimetals Our strategy to synthesize a 3D Dirac SM is as follows. Let us consider a system having both the TRS and IS. In general, the TRS requires E n ,↑ ( k )= E n ,↓ (− k ), where E n , σ ( k ) indicates the energy eigenvalue of the n -th band with the spin σ =↑, ↓ at the momentum k . On the other hand, the IS requires E n , σ ( k )= E n , σ (− k ). Therefore, under the combined operation of TRS and IS, E n ,↑ ( k )= E n ,↓ ( k ), hence, the energy band is doubly degenerate locally at each k . Under this condition, whenever an ABC occurs between the valence and conduction bands, a 3D DP with fourfold degeneracy can be generated. According to Murakami et al . [4] , [5] , [6] , such an ABC can be achieved only under certain limited conditions because of the strong repulsion between degenerate bands. Namely, only when the valence and conduction bands have the opposite parities, an ABC can occur at a TRIM by tuning an external parameter m . In this case, a 3D DP appears at the quantum critical point ( m = m c ) between a normal insulator and a Z 2 topological insulator (see Fig. 1a ). As a band gap opens immediately once m ≠ m c , the DP is unstable. However, in many crystals, the rotational symmetry as well as TRS and IS presents ubiquitously and constrains the physical properties of materials. Surprisingly, as we will describe in detail below, the additional uniaxial rotational symmetry strongly modifies the condition for ABC, which allows the 3D Dirac SM to emerge as a stable phase. This is possible because when the valence and conduction bands have different rotation eigenvalues, the level repulsion between them can be significantly relaxed as pointed out by Wang et al . [17] , [18] , which eventually leads to the emergence of a stable 3D Dirac SM phase in the wide range of the parameter space (see Fig. 1b, c ). 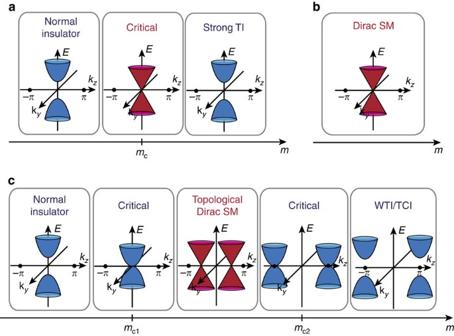Figure 1: Creation of a topological Dirac semimetal via accidental gap closings. (a) The phase transition induced by an accidental band crossing (ABC) when a single control parametermis varied in systems with the TRS and IS but lacking the rotation symmetry. The 3D Dirac fermion appears only at the critical pointm=mcand the ABC mediates the transition between a normal insulator and a strong topological insulator (TI). When an additional uniaxial rotational symmetry is included, two different phase diagrams can be obtained as shown inbandc. Here we choose thekzaxis as the axis for then-fold rotation. (b) The Dirac SM persists irrespective ofm. The Dirac point locates at a TRIM on the rotation axis. The Dirac SM inTable 2corresponds to this case. (c) A stable topological Dirac SM phase appears whenmc1<m<mc2, which mediates the transition between a normal insulator and a weak topological insulator (WTI) or a topological crystalline insulator (TCI). Here a pair of bulk Dirac points, each of which has fourfold degeneracy at the gapless point, exist along the rotation axis and approach the Brillouin zone (BZ) boundary asmincreases. The Dirac SM inTable 1corresponds to this case. At the quantum critical points (m=mc1orm=mc2), the energy dispersion along thekzdirection is quadratic while the dispersion along thekxandkydirections is linear (linear Dirac SM) or quadratic (quadratic Dirac SM) or cubic (cubic Dirac SM). Figure 1: Creation of a topological Dirac semimetal via accidental gap closings. ( a ) The phase transition induced by an accidental band crossing (ABC) when a single control parameter m is varied in systems with the TRS and IS but lacking the rotation symmetry. The 3D Dirac fermion appears only at the critical point m = m c and the ABC mediates the transition between a normal insulator and a strong topological insulator (TI). When an additional uniaxial rotational symmetry is included, two different phase diagrams can be obtained as shown in b and c . Here we choose the k z axis as the axis for the n -fold rotation. ( b ) The Dirac SM persists irrespective of m . The Dirac point locates at a TRIM on the rotation axis. 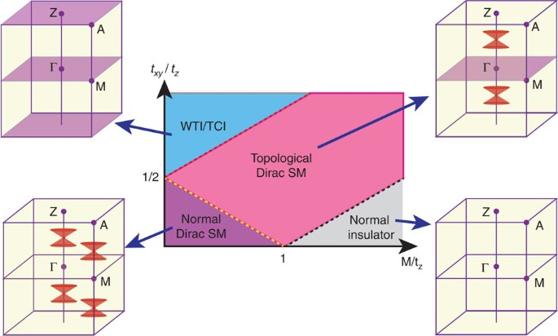Figure 2: Phase diagram. Generic phase diagram of the system with the time-reversal, inversion and rotation symmetries. It is obtained by numerically solving the lattice Hamiltonians in equations (16) and (19), both of which lead to the same phase diagram. HereMindicates the on-site energy difference between two orbitals andtxy(tz) describes the hopping amplitude along the direction perpendicular (parallel) to the rotation axis. For each phase, the location of the 3D bulk Dirac point in the first BZ, if it is present, is indicated by the red symbol having the shape of a Dirac cone. When the two-dimensional (2D) plane withkz=0 orkz=πpossesses a nontrivial 2D topological invariant, such asZ2invariant (ν2D) or the mirror Chern number (nM), the corresponding plane is coloured in purple. If any of these 2D planes carries a non-zero 2D topological invariant, the surface of the material, which is parallel to the axis of the rotation, supports 2D surface Dirac cones. In the figure, WTI and TCI indicate a weak topological insulator and a topological crystalline insulator, respectively. A gap-closing happens at the Γ (Z) point on the black (red) dotted line, whereas a gap-closing occurs at theMpoint on the yellow dotted line. The Dirac SM in Table 2 corresponds to this case. ( c ) A stable topological Dirac SM phase appears when m c1 < m < m c2 , which mediates the transition between a normal insulator and a weak topological insulator (WTI) or a topological crystalline insulator (TCI). Here a pair of bulk Dirac points, each of which has fourfold degeneracy at the gapless point, exist along the rotation axis and approach the Brillouin zone (BZ) boundary as m increases. The Dirac SM in Table 1 corresponds to this case. At the quantum critical points ( m = m c1 or m = m c2 ), the energy dispersion along the k z direction is quadratic while the dispersion along the k x and k y directions is linear (linear Dirac SM) or quadratic (quadratic Dirac SM) or cubic (cubic Dirac SM). Full size image To describe an ABC of two bands, each of which is doubly degenerate because of the simultaneous presence of TRS and IS, a 4 × 4 matrix Hamiltonian can be used as a minimal Hamiltonian, which in general has the following form, where the Pauli matrix σ 1,2,3 ( τ 1,2,3 ) indicates the spin (orbital) degrees of freedom and σ 0 and τ 0 are the 2 × 2 identity matrices. h σσ ′ ( σ , σ ′=↑, ↓) indicates a 2 × 2 matrix, which can be spanned by τ 0,1,2,3 and a ij ( k ) are real functions of k . The invariance of the system under the C n rotation (the n -fold rotation about a principle axis) gives , where R n is the 3 × 3 rotation matrix defining the 2 π / n rotation in the 3D space [21] . Without loss of generality, we can choose the k z axis as the axis of the C n rotation. Then along the k z axis on which R n k = k is satisfied, [ C n , H ( k )]=0. Therefore, we can choose a basis in which both and C n are diagonal, hence, all bands on the k z axis can be labelled by the corresponding eigenvalues of C n . In such a basis, the Hamiltonian can be written as , where d 0,1,2,3 ( k z , m ) are real functions. As the simultaneous presence of TRS and IS requires the double degeneracy of each state, among d 1,2,3 , only one function can be non-zero. Also, as the degenerate bands should have the opposite spin directions, d 1 =0. Hence, the Hamiltonian becomes , where Γ is either Γ= τ 3 or Γ= σ 3 τ 3 . Then, as the energy gap is given by 2| d ( k z , m )|, an ABC can be achieved if and only if d ( k z , m )=0. Here the number of variables (two) is larger than the number of equations (one) to be satisfied for the band crossing, hence, the Dirac SM can always be created via an ABC. Moreover, owing to the TRS and IS, d ( k z ) has a definite parity under the sign reversal of k z as shown in Methods. In fact, the parity of d ( k z ) can be simply determined by the matrix representation P of the IS. Namely, when P has a diagonal form such as P =± τ 0 or ± τ z , d ( k z ) is even, whereas it is odd if P has an off-diagonal form P =± τ x . At first, when d ( k z ) is even, in the leading order with constants M and t z . In this case, the system is a gapped insulator (a Dirac SM) when Mt z >0 ( Mt z <0). Namely, by taking M as a tunable parameter and assuming t z <0, the transition from an insulator ( M <0) to a 3D Dirac SM ( M >0) can be achieved across the sign reversal of M (or the band inversion). In particular, the 3D Dirac SM phase possesses two DPs, which are symmetrically located with respect to the centre of the rotation axis at . The Dirac SMs realized in Cd 3 As 2 and Na 3 Bi belong to this class [17] , [18] . On the other hand, when d ( k z ) is odd, d ( k z )≈ ʋk z in the leading order with a constant ʋ . In this case, there is a single 3D DP at k z =0. Then the system is nothing but a stable 3D Dirac SM with a single DP at the centre of the rotation axis. Considering the full periodic structure of the Brillouin zone (BZ), both k z =0 and k z = π , that is, the TRIMs on the rotation axis, are the possible locations of the DP. The candidate Dirac SM systems such as β-cristobalite BiO 2 (ref. 15 ) and distorted spinels [16] proposed by the recent theoretical studies belong to this class. In these systems, P =± τ x representation is realized due to the non-symmorphic space group symmetry of the system with two sublattice degrees of freedom. Namely, the system is invariant under the inversion with respect to a lattice site followed by a partial translation between sublattice sites. As the sublattices are interchanged through the symmetry operation, P can have an off-diagonal form of P =± τ x . In distorted spinels, the compound IS combined with additional twofold rotation and time-reversal symmetries gives rise to a single DP at the T point of the BZ [16] . On the other hand, there are three bulk DPs in β-cristobalite BiO 2 at the three symmetry-related X points [15] . At each X point, the system has a uniaxial fourfold rotation symmetry with the compound IS P consistent with our theory. In conclusion, when the material has the TRS, IS and uniaxial rotation symmetry simultaneously, there are two different ways to obtain a stable Dirac SM phase. One is through an ABC (or a band inversion), which gives rise to a stable 3D Dirac SM with a pair of 3D DPs on the axis of the rotation (see Fig. 1c ). This class of Dirac SMs appears when the IS is represented by P =± τ 0 or ± τ z . The other case is when the system naturally supports a 3D DP at a TRIM on the rotation axis due to the symmetry of the system (see Fig. 1b ). Such a Dirac SM can exist when the IS is represented by P =± τ x . The intrinsic properties of the relevant 3D Dirac SM phases are summarized in Tables 1 and 2 , respectively. Up to now, we have considered only the leading order terms of d ( k z ). However, when the higher order terms are included, the number of DPs can be increased as a pair of DPs can always be created whenever an additional ABC happens. However, independent of the total number of DPs, the Dirac SM with P =± τ 0, z always has an even number of DPs away from the TRIM, whereas the Dirac SM with P =± τ x having an odd number of DPs always possesses a single DP at a TRIM. Table 1 Classification table for 3D topological Dirac semimetals. Full size table Table 2 Classification table for 3D Dirac SMs with a single Dirac point. Full size table Classification table The classification of the 3D Dirac SM phases can be performed rigorously by imposing the TRS, IS and C n rotation symmetry to the minimal 4 × 4 Hamiltonian H ( k ). In the simultaneous presence of the TRS and IS, the Hamiltonian can always be written as , where Γ i indicates 4 × 4 hermitian matrices satisfying {Γ i , Γ j }=2 δ ij , which guarantees the double degeneracy of eigenstates at each k (see Methods). The precise functional form of a i ( k ) can be fixed by imposing the C n rotational symmetry using the basis under which both C n and H ( k ) are diagonal along the k z direction [21] . The results of the complete classification are concisely summarized in Tables 1 and 2 . Because of the TRS, the rotation operator becomes , where each component u can be written as with p =0,1,..., n −1 and A , B indicate the orbital degrees of freedom. Hence, only two components of C n are independent. The properties of the 3D Dirac SM generated via ABCs are shown in Table 1 . In general, the ABC requires the valence and conduction bands to have different C n eigenvalues. Namely, { u A ,↑ , u A ,↓ } and { u B ,↑ , u B ,↓ } should not have common elements to avoid interband hybridization. However, in the case of C 2 invariant systems, { u A ,↑ , u A ,↓ }={ u B ,↑ , u B ,↓ }={ i , − i }, hence, the ABC is not allowed. On the other hand, the systems with C 3 , C 4 and C 6 symmetries can support 3D Dirac SM phases. Although the detailed structure of the Hamiltonian H ( k ) depends on the specific symmetries of the corresponding system, there are only two different types of low-energy effective Hamiltonians near the bulk gap-closing point. In the first case, after some suitable unitary transformations, the effective Hamiltonian near each of the bulk DP can be written as where the momentum q is measured with respect to the DP. This is the Hamiltonian for the conventional Dirac fermion (the linear Dirac fermion), which is composed of two Weyl fermions having the Chern number +1 or −1, respectively. Whereas in the case of the C 6 invariant system with the , the effective Hamiltonian is given by Note that this DP is composed of two double-Weyl fermions, which have the Chern number +2 or −2, respectively [21] , [22] . Hence, we call this gapless fermions as the quadratic Dirac fermions. The physical properties of the 3D Dirac SM with a DP at the centre of the rotation axis are summarized in Table 2 . As the IS flips the orbitals in this case ( P =± τ x ), the doubly degenerate states at each momentum on the k z axis have different orbitals and opposite spin directions. Therefore, the band crossing between degenerate bands requires { u A ,↑ , u B ,↓ }∩{ u B ,↑ , u A ,↓ }= contrary to the previous case. Moreover, owing to the additional constraint of u A ,↑ =− u B ,↑ , the Dirac SM phase with a single DP cannot exist in the system with C 3 invariance, whereas the systems with C 2 , C 4 , C 6 symmetries support it (see Methods). One interesting prediction of Table 2 is that when the system has C 6 symmetry with , the low-energy Hamiltonian near the DP can be written as Note that this DP is composed of two triple-Weyl fermions, which have the Chern number +3 or −3, respectively [21] . Hence, we can call this gapless fermion as the cubic Dirac fermion. For the other cases in Table 2 , the effective Hamiltonian near the DP is simply described by the ordinary linear Dirac fermions. Topological properties of the 3D Dirac semimetals One important characteristic of the 3D Dirac SM generated by an ABC is that it carries a quantized topological invariant although it is a gapless SM. In fact, the band inversion associated with the ABC is the common origin of the presence of the 2D topological invariant and the emergence of bulk DPs. As shown in Table 1 , in each case, a quantized 2D topological invariant can be defined on the k z =0 plane where the ABC occurs. First of all, as the k z =0 plane can be considered as a 2D system with TRS, a 2D Z 2 invariant ν 2D is well-defined on it [23] , [24] . Moreover, because of the simultaneous presence of the TRS and IS, ν 2D can be determined by the parities of the occupied bands at TRIM [25] . Therefore, when the valence and conduction bands have the opposite parities ( P =± τ z ), the band inversion on the k z =0 plane, which generates a pair of bulk DPs, changes ν 2D by 1, that is, Δ ν 2D =1. This can be contrasted to the case when two bands have the same parity ( P =± τ 0 ), in which Δ ν 2D =0. On the other hand, the presence of additional crystalline symmetries allows us to introduce new topological invariants [26] , [27] , [28] . In particular, when the system has either C 4 or C 6 symmetry, the k z =0 plane carries an integer topological invariant (the mirror Chern number) because of the mirror symmetry of the system [29] , [30] . Here the mirror symmetry appears because of the simultaneous presence of the π rotation ( R π ) with respect to the k z axis and the IS. Then, the combined operation of the IS and π rotation defines the mirror symmetry M = PR π , which connects the Hamiltonian H ( k x , k y , k z ) and H ( k x , k y , − k z ), hence, the system is invariant under the mirror symmetry ( M ) in the k z =0 plane. As M 2 =−1, the Hamiltonian can be block-diagonalized with each block characterized by the mirror eigenvalue ± i , respectively. Then, the Chern number can be defined in each block ( C ± i ), separately. Although the total Chern number C + i + C − i =0 because of the TRS, the difference (the mirror Chern number) can be non-zero. Note that R π exists only in systems with the C 4 or C 6 symmetry with the corresponding or , respectively. Therefore, the C 3 invariant system is characterized only by the 2D Z 2 invariant ν 2D , whereas the system with the C 4 or C 6 symmetry has both the Z 2 invariant ν 2D and the mirror Chern number n M , where n M and ν 2D are equivalent up to the modulo 2. In Methods, we have described how the mirror symmetry manifests in the system in terms of the effective Hamiltonian H ( k ). When either ν 2D or n M is non-zero, the 3D Dirac SM supports 2D surface Dirac cones when a surface parallel to the k z axis is introduced. The number of 2D Dirac cones on one surface is given by | n M | (| ν 2D |) when the system has the C 4 or C 6 ( C 3 ) symmetry. Lattice model and generic phase diagram Let us illustrate the intriguing properties of the 3D topological Dirac SM phases in Table 1 by studying lattice Hamiltonians numerically. For convenience, we choose the C 4 invariant systems with P = τ 0 or P = τ z corresponding to the 6th or 7th row of Table 1 , respectively. However, the main features of the phase diagram can be applied to all cases in Table 1 because the overall structure of the phase diagram is solely determined by the single function a 5 ( k ), whose leading order functional form is the same in all cases. The detailed information about the lattice Hamiltonian is presented in Methods. Figure 2 summarizes the main properties of the lattice Hamiltonian. In general, the system supports four different phases as shown in the phase diagram. The phase transition is always accompanied by an ABC on the k z =0 or k z = π plane, in which a pair of 3D bulk DPs are either created or annihilated. Whenever an ABC happens, it also changes the 2D topological invariant of the corresponding 2D planes. Figure 2: Phase diagram. Generic phase diagram of the system with the time-reversal, inversion and rotation symmetries. It is obtained by numerically solving the lattice Hamiltonians in equations (16) and (19), both of which lead to the same phase diagram. Here M indicates the on-site energy difference between two orbitals and t xy ( t z ) describes the hopping amplitude along the direction perpendicular (parallel) to the rotation axis. For each phase, the location of the 3D bulk Dirac point in the first BZ, if it is present, is indicated by the red symbol having the shape of a Dirac cone. When the two-dimensional (2D) plane with k z =0 or k z = π possesses a nontrivial 2D topological invariant, such as Z 2 invariant ( ν 2D ) or the mirror Chern number ( n M ), the corresponding plane is coloured in purple. If any of these 2D planes carries a non-zero 2D topological invariant, the surface of the material, which is parallel to the axis of the rotation, supports 2D surface Dirac cones. In the figure, WTI and TCI indicate a weak topological insulator and a topological crystalline insulator, respectively. A gap-closing happens at the Γ ( Z ) point on the black (red) dotted line, whereas a gap-closing occurs at the M point on the yellow dotted line. Full size image There are two different types of insulators in the phase diagram. One is a normal insulator, which does not carry a topological number, and the other is either a weak topological insulator or a topological crystalline insulator, in which both the k z =0 and k z = π planes have nontrivial 2D topological invariants. The system with P =± τ z supports a weak topological insulator, which has the Z 2 topological index of ( ν 0 ; ν 1 ν 2 ν 3 )=(0; 001) because ν 2D =1 in both the k z =0 and k z = π planes. On the other hand, when P =± τ 0 , ν 0,1,2,3 =0 independent of the band inversion because every band has the same parity. However, it is possible to obtain a topological crystalline insulator, as both the k z =0 and k z = π planes can have the non-zero mirror Chern number of n M =2. In fact, it is to note that the weak topological insulator in the system with P =± τ z can also have finite mirror Chern numbers. However, for convenience, we mainly focus on the Z 2 invariant to characterize the system with P =± τ z . The 3D Dirac SM phases can also be distinguished in two different ways. At first, when the Dirac SM phase has a non-zero topological invariant in either the k z =0 plane or the k z = π plane, we can call it a topological Dirac SM as the Dirac SM carries stable 2D Dirac cones on the surface. Similarly, a topologically trivial Dirac SM can be defined when the system does not have any topological invariant in both planes. However, in both cases, independent of the presence of the 2D topological invariants, the 3D Dirac SM phase is stable because the symmetry of the system and occupies a finite region in the phase diagram. 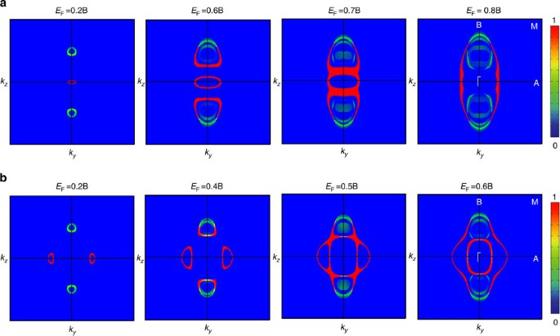Figure 3: Evolution of the Fermi surface of a [100] film varying the Fermi energy. The wave function amplitudes confined within the first five layers from the top surface are plotted for the states touching the Fermi level (EF). To obtain the Fermi surface we have solved numerically the lattice Hamiltonian in equations (16) and (19). (a) For a topological Dirac semimetal withC4symmetry, which hasν2D=1 on thekz=0 plane. The closed loop at the centre of the surface BZ is from a 2D surface Dirac point at the Γ point. Two 3D bulk Dirac cones also produce finite intensity symmetrically on thekzaxis. AsEFincreases, the closed loop due to the 2D Dirac point deforms to a pair of Fermi arcs connected to the bulk states. (b) For a topological Dirac semimetal withC4symmetry, which hasnM=2 on thekz=0 plane. The two closed loops on thekyaxis are due to two 2D Dirac points localized on the surface. AsEFincreases, the closed loops due to 2D Dirac cones turn into four Fermi arcs. In bothaandb, the 3D bulk Dirac fermions show the linear dispersion in the momentum space. Hence, the number of surface Fermi arcs is solely determined by the 2D topological invariant on thekz=0 plane independent of the dispersion of the bulk Dirac fermions. Figure 3 shows the evolution of the Fermi surface of the topological Dirac SM system with a slab geometry whose surface normal is parallel to the [100] direction. The translational symmetry of the system in the yz plane is maintained. Here we first pick the states touching the Fermi level ( E F ) and then plot the wave function amplitudes of the corresponding state localized on the first five layers from the top surface. The red colour indicates the states localized on the [100] surface, whereas the bright blue colour corresponds to the 3D bulk Dirac states. In the case of the topological Dirac SM with ν 2D =1 in the k z =0 plane, a 2D surface Dirac cone appears on the k y axis centred at the Γ point as shown in Fig. 3a . Here the two bulk DPs give rise to the finite intensity on the k z axis located symmetrically with respect to the Γ point. When the Fermi energy ( E F ) is near the bulk DP ( E F =0 at the DP), the bulk and surface states are decoupled, and the surface states form an isolated closed loop. As E F increases, the Fermi surface topology evolves continuously, and when the bulk and surface states start to overlap, the 2D surface state is deformed to the Fermi arc structure. Namely, the Fermi arcs of 3D Dirac SM emerge simply because of the deformation of the 2D Dirac cone, which exists due to the fact that ν 2D =1 on the k z =0 plane. As such an evolution of the surface spectrum occurs continuously, the Fermi arc states can appear even when E F =0 if the parameters of the model Hamiltonian are tuned properly. Figure 3: Evolution of the Fermi surface of a [100] film varying the Fermi energy. The wave function amplitudes confined within the first five layers from the top surface are plotted for the states touching the Fermi level ( E F ). To obtain the Fermi surface we have solved numerically the lattice Hamiltonian in equations (16) and (19). ( a ) For a topological Dirac semimetal with C 4 symmetry, which has ν 2D =1 on the k z =0 plane. The closed loop at the centre of the surface BZ is from a 2D surface Dirac point at the Γ point. Two 3D bulk Dirac cones also produce finite intensity symmetrically on the k z axis. As E F increases, the closed loop due to the 2D Dirac point deforms to a pair of Fermi arcs connected to the bulk states. ( b ) For a topological Dirac semimetal with C 4 symmetry, which has n M =2 on the k z =0 plane. The two closed loops on the k y axis are due to two 2D Dirac points localized on the surface. As E F increases, the closed loops due to 2D Dirac cones turn into four Fermi arcs. In both a and b , the 3D bulk Dirac fermions show the linear dispersion in the momentum space. Hence, the number of surface Fermi arcs is solely determined by the 2D topological invariant on the k z =0 plane independent of the dispersion of the bulk Dirac fermions. Full size image The energy spectrum of the topological Dirac SM with n M =2 on the k z =0 plane also shows a similar variation as described in Fig. 3b . As n M =2, there are two 2D surface Dirac cones on the k y axis. As E F increases, the surface Dirac cones evolve to Fermi arcs when the surface and bulk states overlap. As the number of surface Dirac cones is two, the number of surface Fermi arc is also doubled as compared with the case shown in Fig. 3a . It is worth to note that in both cases shown in Fig. 3a,b , the energy dispersion near the bulk 3D DP is basically the same, that is, the bulk state shows the linear dispersion relation in all three momentum directions. This clearly shows that the number of Fermi arcs of the topological Dirac SM is irrespective of the dispersion of the bulk states. It is worth to stress that the physical origin of the surface Fermi arcs in the 3D Dirac SM is clearly distinct from that of the Weyl SM which has twofold degeneracy at the gap-closing point. In the Weyl SM, the Chern number carried by the bulk gapless point (Weyl point) guarantees the emergence and stability of the Fermi arc states [31] , [32] , [33] . As the Chern number of the Weyl point is purely determined by the energy dispersion around the Weyl point, the number of Fermi arcs in the system with a fixed number of Weyl points strongly depends on the energy dispersion near the Weyl point. In conventional Weyl SMs with the linear dispersion around the Weyl point, the number of Fermi arcs on one surface of the sample is equal to the number of Weyl point pairs in the first BZ. On the other hand, in the case of Weyl SMs with double (triple)-Weyl fermions whose dispersion is quadratic (cubic) along the two momentum directions but linear in the third direction, the number of Fermi arcs is double (triple) of the number of the Weyl point pairs [21] , [22] . However, in contrast to the case of the Weyl SM, the physical origin of the surface states of the 3D Dirac SM is independent of the energy dispersion of the 3D bulk Dirac fermions. Because of the simultaneous presence of the TRS and IS, the Chern number of each 3D DP is zero. Here the number of the Fermi arcs on the surface of the sample is solely determined by the 2D topological invariant on the k z =0 (or k z = π ) plane irrespective of the energy dispersion around the 3D DP. Therefore, although the low-energy Hamiltonian near the 3D bulk DP is the same, the number of Fermi arcs can be different depending on the 2D topological invariant of the system as shown above. Up to now, we have considered the system with a uniaxial rotation symmetry together with TRS and IS. As most crystals have a larger symmetry with multiple rotation axes, it is important to understand how our theory can be applied to these systems. First of all, it is worth to note that the location of the two DPs can be anywhere on the rotation axis in the case of the Dirac SMs with P =± τ 0, z in Table 1 . Therefore, the primary rotation axis should be the line connecting the two DPs in this case. Even if there are multiple pairs of DPs in the BZ, we can easily specify the primary rotation axis for each pair of DPs by using the fact that the centre of the rotation axis locates at a TRIM and the relative orientation of different rotation axes should satisfy the crystalline symmetry. Once the primary rotation axis is specified, we can apply our classification scheme to each pair of DPs. On the other hand, in the case of the Dirac SM with P =± τ x in Table 2 , the role of the additional crystalline symmetry is more significant because the DP locates at a TRIM where the system generally has a higher crystalline symmetry. At this point, it is useful to note that the threefold rotation symmetry prohibits a DP at a TRIM according to Table 2 . In fact, this imposes a strong constraint to the allowed position of the DP, and we can rule out the Γ point as a possible location of the DP because the space groups allowing the fourfold degeneracy at the Γ point always have a threefold rotation symmetry (see Methods and also ref. 15 ). Therefore, a DP can locate only at a TRIM on the BZ surface. Even if the point group symmetry of the crystal contains many rotation axes, the symmetry on the BZ surface can be much lower and the system often has a uniaxial rotation symmetry at a TRIM on the BZ surface. For example, in both β-cristobalit BiO 2 and distorted spinels, there is a uniaxial rotation symmetry at the momentum where each DP presents. In this situation, it is straightforward to apply our theory. To sum up, although the point group symmetry of the crystal has multiple rotation axes, the local symmetry at the momentum where each DP presents is much lower, hence, our theory can be applied to crystalline solids in general. We conclude with a discussion about the stability of the 3D Dirac SM under the influence of the Coulomb interaction and disorder. Simple power counting shows that the long-range Coulomb interaction is a marginally irrelevant perturbation to the 3D Dirac fermions with the linear dispersion [34] , [35] , [36] . Hence, various physical properties of the 3D Dirac SM can receive logarithmic corrections because of the long-range Coulomb interaction similar to the cases of 3D Weyl SM [35] , [36] , [37] and graphene [38] , [39] , [40] . On the other hand, as the disorder is irrelevant according to the power counting, we expect the Dirac SM state can be stable at least against weak disorder effect. However, as the crystalline symmetry is important for the protection of the DP, strong disorder can induce nontrivial physical consequences to 3D Dirac SM phase, especially when the interaction and disorder effect are considered simultaneously [34] . Moreover, in the case of the quadratic Dirac SM and the cubic Dirac SM, the effect of the interaction and disorder can be more significant. As the in-plane dispersion becomes either quadratic or cubic in the momentum space, which strongly enhances the low energy density of states, it is expected that the interaction and disorder can even bring about new exotic quantum phases. For instance, according to a recent theoretical study, an exotic non-Fermi liquid state can appear in a 3D SM having quadratic energy dispersion in the momentum space [41] . As the interplay between the long-range Coulomb interaction and nontrivial screening because of the enhanced low energy density of states is the fundamental origin leading to the non-Fermi liquid phase, the quadratic Dirac SM and the cubic Dirac SM are also promising systems to observe novel quantum critical states. Finally, let us note that the quantum critical point in Fig. 1c where the pair creation or pair annihilation of bulk DPs happens is another interesting venue to observe a new types of quantum critical phenomena. At the quantum critical point, as the energy dispersion along the rotation axis is always quadratic, the low-energy excitation can show highly anisotropic dispersion relations in the linear Dirac SM and cubic Dirac SM. According to the recent theoretical study [42] , [43] , it is shown that such an anisotropic dispersion can induce a novel screening phenomenon, which can induce anomalous distribution of the screening charge around a charged impurity. To reveal the fascinating physical properties of the linear Dirac SM and the triple Dirac SM at the critical point would be another interesting topic for future studies. The classification procedure The classification of the minimal 4 × 4 matrix Hamiltonian H ( k ) can be performed as follows. At first, let us impose the TRS on H ( k ). The TRS can be represented by the operator Θ= iσ y K , where σ x , y , z are Pauli matrices for spin degrees of freedom and K stands for complex conjugation. The invariance of the Hamiltonian under TRS, that is, H (− k )=Θ H ( k )Θ −1 gives rise to the relations and , where the superscript T indicates the transposition. Then, the resulting Hamiltonian with the TRS can be written in the following way. where the superscript * indicates the complex conjugation. Second, to impose the IS on the Hamiltonian H ( k ), we have to determine the matrix representation P of the IS. As the IS is independent of the spin-rotation, in general, , where indicate the Pauli matrices for orbital degrees of freedom and p 0, x , y , z are complex numbers. As the operation of P 2 relates the same electronic states, it should be equivalent to the identity operator up to a global U(1) phase factor, that is, . Therefore, P should be either P =± e iφ or , where . To determine φ and , the following three relations can be used: (i) [ T , P ]=0, (ii) P † P =1 and (iii) ( TP ) 2 =−1. Then, the general solution for P is given by P =± τ 0 or P =cos θτ z −sin θτ x with θ ε[0,2 π ]. The invariance of the Hamiltonian under P , that is, H (− k )= PH ( k ) P −1 combined with the TRS constrains the possible form of the Hamiltonian, which can be summarized in the following way. (i) When P =± τ 0 . , where Γ 1 = τ x , Γ 2 = τ y σ z , Γ 3 = τ y σ x , Γ 4 = τ y σ y , Γ 5 = τ z . Hence, h ↑↑ = a 0 + a 1 τ x + a 2 τ y + a 5 τ z and h ↑↓ =( a 3 − ia 4 ) τ y . Here a 0,1,2,3,4,5 ( k ) are all real and even under the sign change of k . (ii) When P =cos θτ z −sin θτ x . , where Γ 1 = μ x σ z , Γ 2 = μ y , Γ 3 = μ x σ x , Γ 4 = μ x σ y , Γ 5 = μ z and all a 0,1,2,3,4,5 are real functions. Hence, h ↑↑ = a 0 + a 1 μ x + a 2 μ y + a 5 μ z and h ↑↓ =( a 3 − ia 4 ) μ x . Here a 0,5 (− k )= a 0,5 ( k ), a 1,2,3,4 (− k )=− a 1,2,3,4 ( k ) and μ x =cos θτ x +sin θτ z , μ y = τ y , μ z =−sin θτ x +cos θτ z . In both cases, an ABC is possible only if the five equations a 1,2,3,4,5 =0 are satisfied simultaneously. Here each function a i has four variables including the three momentum components k x , y , z and one external control parameter m , that is, a i = a i ( k x , k y , k z , m ). As the number of equations to be satisfied is five, whereas the number of variables is four, the condition for the ABC cannot be satisfied in general at a generic momentum k . However, it is worth to note that the above consideration does not rule out the ABC at non-generic points in the momentum space with high symmetry. For instance, as pointed out by Murakami [4] , at the time-reversal invariant momentum k = k TRIM , where k and − k are equivalent, all odd functions in H ( k ) vanish. In the case of (ii) with P =cos θτ z −sin θτ x , a 1,2,3,4 ( k TRIM )=0. Therefore, an ABC is possible if and only if one condition a 5 ( k TRIM , m )=0 is satisfied, which can be achieved by tuning one external control parameter m . This is the reason why the topological phase transition between two insulators can occur through an ABC at a time-reversal invariant momentum. Now let us show how the condition for ABC is modified by the presence of the additional rotation symmetry C n with respect to the z axis. Here n is restricted to be n =2,3,4,6 in periodic lattice systems. Using a basis in which both and C n are diagonal, C n can be represented by a diagonal matrix C n =diag[ u A ,↑ , u B ,↑ , u A ,↓ , u B ,↓ ]=diag[ α p , α q , α r , α s ], where with p =0, 1, ..., n −1 (ref. 21 ). For convenience, we express C n in the following way: The invariance of the Hamiltonian under C n leads to where k ± = k x ± ik y . From equation (1), we can obtain that The equations above can be further simplified by considering the constraint on C n because of TRS. Namely, as [ T , C n ]=0, we can show that , and . Namely, . Then equation (2) becomes In general, h ↑↑ ( k ) and h ↑↓ ( k ) can be represented by where f 0, z are real functions, whereas f + , g 0± z are complex functions. Also τ ± = τ x ± iτ y . As f 0 does not affect the gap-closing, we can neglect it in the forthcoming discussion. Equation (3) gives the following relations: and where g 0± z = g 0 ± g z . The equations (5) and (6) are the key results, which lead to the full classification of the 3D Dirac SM. For the classification, we first consider the TRS and IS, which restrict the possible structure of the Hamiltonian summarized in (i) and (ii). After that the rotational symmetry is imposed to the Hamiltonian by using the equations (5) and (6). As shown previously, the most general form of P is given by P =± τ 0 or P =cos θτ z −sin θτ x with θ ε[0, 2 π ]. To determine the matrix representation of P and C n , we use the basis in which both the and C n are diagonal. As noted before, in such a basis, the Hamiltonian should have a diagonal form given by with Γε{ τ z , τ z σ z }. As d ( k z ) should have a definite parity under IS as shown in (i) and (ii), the possible form of P is restricted to be P =± τ 0 , ± τ x , ± τ z . In particular, when P =± τ 0 or ± τ z , d ( k ) is even under the sign change of the momentum k , which leads to the 3D topological Dirac SM via an ABC as summarized in Table 1 . On the other hand, when P =± τ x , d ( k ) is odd under the sign change of k , which gives rise to a 3D Dirac SM with a single bulk DP as summarized in Table 2 . Let us describe the constraints from the rotation symmetry in detail. When P =± τ 0 , the Hamiltonian h ↑↑ ( k ) and h ↑↓ ( k ) are given by On the other hand, when P =± τ z , In both cases, fromequations (5) and (6), we can obtain where f + ( k )=( a 1 ( k )− ia 2 ( k ))/2 and g ( k )=( a 3 ( k )− ia 4 ( k ))/2. As f + and g should be zero on the k z axis, we obtain and . Hence, the ABC is possible when { u A ,↑ , u A ,↓ }∩{ u B ,↑ , u B ,↓ }= , that is, when the valence and conduction bands have no rotation eigenvalue in common. Finally, when P =± τ x , the Hamiltonian h ↑↑ ( k ) and h ↑↓ ( k ) are given by From the equations (5) and (6), we can obtain where f + ( k )=( a 5 ( k )− ia 2 ( k ))/2 and g z ( k )=( a 3 ( k )− ia 4 ( k )). From the condition that f + = g z =0 on the k z axis, we obtain , , and . Namely, the following two conditions should be satisfied: The physical meaning of these two conditions is as follows. First of all, as the IS flips the orbitals in this case ( P =± τ x ), E A , σ ( k z )= E B , σ (− k z ). Then, the combined operation of the TRS and IS ensures E A ,↑ ( k z )= E B ,↓ ( k z ) and E A ,↓ ( k z )= E B ,↑ ( k z ) on the k z axis. Note that the orbital index is physically meaningful in this case, because the angular momentum is a good quantum number on the k z axis. Then, the crossing between two degenerate bands requires { u A ,↑ , u B ,↓ }∩{ u B ,↑ , u A ,↓ }= . Moreover, as ( C n P ) 2 =( PC n ) 2 on the k z axis, C n P =± PC n . However, as the equation (12) is violated if [ C n , P ]=0 is fulfilled, we obtain { C n , P }=0, which immediately leads to the equation (13). In fact, the condition u A ,↑ =− u B ,↑ means with integers p and q . But this relation cannot be satisfied if n =3. Therefore, the 3D Dirac SM with a single DP cannot exist in systems with C 3 invariance. Absence of the symmetry-protected Dirac point at the Γ point Let us explain why the symmetry-protected DP cannot exist at the Γ point in the first BZ. Here we only consider the fourfold degenerate DP, which splits into two doubly degenerate states away from the band crossing point. At the Γ point, the representation of the space group is equivalent to the representation of the point group, which is true for both the non-symmorphic and symmorphic space groups. As the symmetry-protected DP can appear when the space group symmetry at a given momentum allows a four-dimensional irreducible representation, what we have to do is to check the presence of the four-dimensional irreducible representation in the double-valued representation of the relevant point group. It is straightforward to confirm that among the 32-point groups, only the cubic groups T d , O , O h support a four-dimensional irreducible representation in their double-valued representation [44] . However, all these cubic groups contain threefold rotation axes. According to Table 2 , an isolated symmetry-protected DP locating at a TRIM is forbidden if the system has a threefold rotation symmetry. Therefore, we conclude that the symmetry-protected DP cannot present at the Γ point in 3D periodic electronic systems. A similar conclusion is also obtained in ref. 15 . The emergence of the mirror symmetry in the Hamiltonian Let us briefly describe how the mirror symmetry manifests in the effective Hamiltonian . As shown in Table 1 , in systems with the C 4 or C 6 symmetry, either f ( k ) or g ( k ) becomes zero in the k z =0 plane. Although only the lowest order terms are shown in Table 1 , we can show that the same result holds in all orders. This means that the effective Hamiltonian can be written as in the k z =0 plane. Here are three mutually anti-commuting Gamma matrices. As only three Gamma matrices appear in the Hamiltonian, we can define a conserved quantity satisfying . It is straightforward to show that is equivalent to the mirror operator M in all cases, hence, the system has the mirror symmetry in the k z =0 plane. The lattice Hamiltonians We can construct the lattice Hamiltonians straightforwardly by using the information in Tables 1 and 2 . For instance, for the C 4 invariant system with P =± τ z , that is, 6th row of Table 1 , we can use where η , β, γ, M , t xy , t z are real constants. More explicitly, where . In real space, the Hamiltonian becomes where n indicates the lattice sites and are the unit lattice vectors along x , y , z directions. η indicates the nearest neighbour hopping amplitudes in the xy plane, ( β + γ ) denotes the next nearest neighbour hopping amplitudes in the yz and zx planes, and ( β − γ ) indicates the hopping process along the body-diagonal direction of the cubic lattice. M indicates the on-site potential difference between the A and B orbitals, and t xy ( t z ) describes the hopping amplitude difference in different orbitals along the x , y directions (in the z direction). Similarly, for the C 4 invariant system with P =± τ 0 , that is, the 7th row of Table 1 , we use More explicitly, In real space, the Hamiltonian becomes where ( β + γ ) indicates the nearest neighbour hopping amplitudes in the xy plane, ( β − γ ) (η) denotes the next nearest neighbour hopping amplitudes in the xy ( yz and zx ) planes. M , t xy , t z have the same meaning as above. In both cases, we have chosen η =1, β =2, γ =1, t z =1 while varying M and t xy for the numerical computation. How to cite this article: Yang, B.-J. and Nagosa, N. Classification of stable three-dimensional Dirac semimetals with nontrivial topology. Nat. Commun. 5:4898 doi: 10.1038/ncomms5898 (2014).